High yield exfoliation of two-dimensional chalcogenides using sodium naphthalenide Transition-metal dichalcogenides like molybdenum disulphide have attracted great interest as two-dimensional materials beyond graphene due to their unique electronic and optical properties. Solution-phase processes can be a viable method for producing printable single-layer chalcogenides. Molybdenum disulphide can be exfoliated into monolayer flakes using organolithium reduction chemistry; unfortunately, the method is hampered by low yield, submicron flake size and long lithiation time. Here we report a high-yield exfoliation process using lithium, potassium and sodium naphthalenide where an intermediate ternary Li x MX n crystalline phase (X=selenium, sulphur, and so on) is produced. Using a two-step expansion and intercalation method, we produce high-quality single-layer molybdenum disulphide sheets with unprecedentedly large flake size, that is up to 400 μm 2 . Single-layer dichalcogenide inks prepared by this method may be directly inkjet-printed on a wide range of substrates. Post graphene discovery, single-layered transition-metal dichalcogenides (LTMDs), such as MoS 2 and WS 2 , have attracted great attention as next generation two-dimensional (2D) materials owing to their large intrinsic bandgap [1] , [2] , [3] , [4] , [5] , [6] , [7] , [8] , [9] , [10] , [11] , [12] , [13] , which is particularly attractive in view of the gapless nature of graphene [14] , [15] , [16] . Single-layer MoS 2 has attractive attributes such as a direct bandgap (1.9 eV), large in-plane mobilities (200–500 cm 2 V −1 s −1 ), high current on/off ratios (exceeding 10 8 ), as well as remarkable mechanical and optical properties [17] , [18] . Two-dimensional quantum confinement of carriers can be exploited in conjunction with chemical composition to tune the optoelectronic properties of the metal chalcogenides at the nanoscale. These properties are of great interest for applications in optoelectronic devices such as thin film solar cells, photodetectors, flexible logic circuits and sensors [19] , [20] , [21] , [22] , [23] . Transition-metal chalcogenides (TMC) possessing lamellar structures can serve as hosts for the intercalation of a wide variety of electron-donating species ranging from Lewis base to alkali metals [24] , [25] . One well-known class of intercalatants is the organolithium compounds. MoS 2 can be intercalated with lithium to give the reduced Li x MX n phase (X=Se, S, and so on) with expanded lattice, this can be exfoliated in a second step into single-layer sheets by ultrasound-assisted hydration process [26] , [27] , [28] , [29] . However long lithiation time (for example, 3 days at 100 °C) is typically needed when n -butyl lithium is used as lithiation agent due its inclination to form dimeric, trimeric and higher aggregates, which diffuse slowly into the interlayers in large-sized TMC crystals. Subsequent exfoliation from the lithiated MoS 2 suffers a low yield of single-layer flakes, disintegration into submicron-sized flake, formation of metal nanoparticles and precipitation of Li 2 S [5] , [29] . This has limited the development of solution-processed LTMDs in most applications that demand clean and large-sized flakes. An electrochemical approach has been developed recently to produce single-layer MoS 2 and WS 2 flakes; however, the upward scaling of this process is limited by volumetric resistance in battery-type cells [30] . In such electrochemical cells, 10% acetylene black nanoparticles are typically added to the host materials to reduce volumetric resistance but this creates one problem: carbon nanoparticles are mixed with LTMDs and these contaminants are hard to be dislodged from the surface. Similar to the research directions in solution-processed graphene, there is a clear need to explore new chemistry to make high-quality single-layer LTMDs in high yield. The intercalation of lithium into layered molybdenum disulphide may be described as an ion–electron transfer topotactic reaction. In most reported papers, organolithium reagents were used as intercalating agents because of its solubility in a wide range of solvents and the formation of stoichiometric LiMoS 2 ternary products [26] , [27] , [28] , [29] . Compared with Li ions, other alkali ions such as Na or K were less commonly used in exfoliation chemistry. The ionic radii of Na and K are several times larger than that of Li ions, which means that in principle these ions can expand the lattice in the c -axis direction to a larger extent. More importantly, Na and K intercalation compounds react more violently with water than Li compounds, implying that single-layer TMDs should be exfoliated more efficiently. Intercalation of Na and K can also produce different structural and electronic effect compared with Li due to different coordinative complexation by the host. In Li x MX n , Li is always octahedrally coordinated; however, K and Na can occupy octahedral or trigonal prismatic site. This has important implications electronically due to the metallic to semiconductor properties transition in these compounds. Metal electride solution consisting of Na in concentrated liquid ammonia can be a powerful reducing agent, except that ammonia molecule has a tendency to coordinate with Mo and displace S, this can result in decomposition and segregation of Mo nanoparticles [31] , [32] . In spite of numerous reports that discussed the exfoliation of LTMDs, few of these methods can meet the demand of producing high yield, high purity and large-sized flakes [33] , [34] . Our search for alkali metal adducts lead us to naphthalene, which forms intensely coloured compounds with alkali metals. In sodium naphthalenide (Na + C 10 H 8 − ), for example, the metal transfers an electron to the aromatic system to produce a radical anion which has strong reducing properties. Although sodium naphthalenide was first investigated in 1936 by Scott et al. [35] , the synthetic utility of this alkali metal adduct has not been fully explored. It is interesting to consider whether single-layer LTMDs can be produced by reacting MoS 2 with various alkali metal naphthalenide adduct in a radical anion solution. Motivated thus, we prepare naphthalenide adducts of Li, K and Na and compare the exfoliation efficiency and quality of MoS 2 generated. Using a two-step expansion and intercalation method, we report the production of high-quality single-layer MoS 2 flake sheets with unprecedentedly large flake size, that is, up to 400 μm 2 when the Na adduct was intercalated. Single-layer MoS 2 inks prepared by this method could be directly jet-printed on a wide range of substrate. 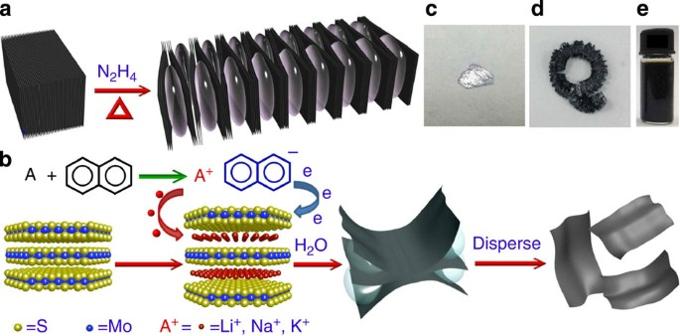Figure 1: Schematic of fabrication processes. (a) Bulk MoS2is pre-exfoliated by the decomposition products of N2H4. (b) Pre-exfoliated MoS2reacts with A+C10H8−to form an intercalation sample, and then exfoliates to single-layer sheets in water. (c) Photograph of bulk single-crystal MoS2, (d) photograph of pre-exfoliated MoS2, (e) photograph of Na-exfoliated single-layer MoS2dispersion in water. Production of LTMDs Figure 1 shows the schematic diagram of the processing steps involved in obtaining well-dispersed samples of LTMDs. First, bulk MoS 2 crystals (or powders) are expanded by reacting with hydrazine (N 2 H 4 ) in hydrothermal condition ( Fig. 1a ). The expansion mechanism can be explained by a redox-rearrangement model in which part of the N 2 H 4 is oxidized to N 2 H 5 + upon intercalation. The intercalated N 2 H 5 + is not thermally stable and will be decomposed to N 2, NH 3 and H 2 upon heating the intercalated MoS 2 films at high temperature. Decomposition and gasification of intercalated N 2 H 4 molecules expands the MoS 2 sheets by more than 100 times compared to its original volume. In a second step, the expanded MoS 2 crystal is intercalated by alkali naphthalenide solution ( Fig. 1b ). Finally the intercalated MoS 2 is exfoliated by dipping in ultrasonicated water operated at low power to avoid fragmentation of the sheets. A black suspension consisting predominantly of 90% single-layer MoS 2 can be obtained after centrifugation and decanting the supernatant ( Supplementary Fig. S1 ). The generic applicability of this method has been tested successfully on a wide range of LTMDs, which includes the high yield exfoliation of monolayer TiS 2 , TaS 2 , and NbS 2 , as well as few layer (2–4) diselenide TiSe 2 , NbSe 2 , and MoSe 2 ( Supplementary Fig. S2 ). Figure 1: Schematic of fabrication processes. ( a ) Bulk MoS 2 is pre-exfoliated by the decomposition products of N 2 H 4 . ( b ) Pre-exfoliated MoS 2 reacts with A + C 10 H 8 − to form an intercalation sample, and then exfoliates to single-layer sheets in water. ( c ) Photograph of bulk single-crystal MoS 2 , ( d ) photograph of pre-exfoliated MoS 2 , ( e ) photograph of Na-exfoliated single-layer MoS 2 dispersion in water. Full size image Intercalation and exfoliation XRD measurements were done on freshly intercalated, hermetically sealed samples after drying in argon and vacuum. The position and intensity of the ( 002 ) peak originating from the hexagonal 2H-MoS 2 can be used to judge the extent of intercalation and exfoliation. In freshly intercalated samples, the ( 002 ) peaks of the pristine MoS 2 is shifted completely toward lower angles, indicating expansion of the lattice along the c -axis and formation of stoichiometric ternary compounds ( Fig. 2 ). The spacing between adjacent layers in the expanded lattice of the each intercalated phase are K c /2=7.92 Å, Na c /2=7.05 Å and Li c /2=6.18 Å, respectively. The increase in the interlayer distance as a result of the intercalation is Δ c /2 =( c /2 - c - c 0 /2), K Δ c /2=1.88 Å, Na Δ c /2 =1.01 Å and Li Δ c /2=0.14 Å. It is worth noting that these Δ c /2 values are much smaller than that of naphthalene-intercalated MoS 2 produced by an exfoliating-restacking process, which indicates that the organic anion is not intercalated in the MoS 2 crystal. Fig. 2b shows that after three days of storage in wet air (humidity around 27.5 g m −3 ), the intensity of the ( 002 ) peaks is reduced and they shift toward smaller angles (K c /2 =8.99 Å, Na c /2 =9.35 and 11.61 Å and Li c /2 =7.08 Å). This additional shift is ascribed to the continuous hydration of the intercalated ions, leading to further lattice expansion. 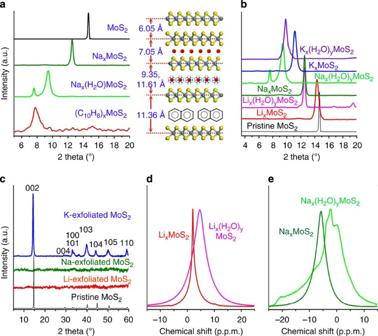Figure 2: Characterization of intercalated and exfoliated MoS2. (a) XRD pattern and schematic of pristine MoS2, Na-intercalated MoS2, after exposure of Na-intercalated MoS2to the ambient for 3 days, exfoliated-and-restacked naphthalene-intercalated MoS2. (b) Li-, Na- and K-intercalated MoS2, after exposure of intercalated sample to the ambient for 3 days. (c) Li-, Na- and K-exfoliated MoS2without any annealing. (d) Solid-state7Li NMR spectra of LixMoS2and Lix(H2O)yMoS2, (e) Solid-state23Na NMR spectra of NaxMoS2and Nax(H2O)yMoS2. Figure 2: Characterization of intercalated and exfoliated MoS 2 . ( a ) XRD pattern and schematic of pristine MoS 2 , Na-intercalated MoS 2 , after exposure of Na-intercalated MoS 2 to the ambient for 3 days, exfoliated-and-restacked naphthalene-intercalated MoS 2 . ( b ) Li-, Na- and K-intercalated MoS 2 , after exposure of intercalated sample to the ambient for 3 days. ( c ) Li-, Na- and K-exfoliated MoS 2 without any annealing. ( d ) Solid-state 7 Li NMR spectra of Li x MoS 2 and Li x (H 2 O) y MoS 2 , ( e ) Solid-state 23 Na NMR spectra of Na x MoS 2 and Na x (H 2 O) y MoS 2 . Full size image The intercalated compounds are exfoliated by hydration, and the exfoliated sheets are dried into powder form and characterized by XRD ( Fig. 2c ). In the case of K-intercalated MoS 2 , peaks due to the intercalated host compound as well as restacked ( 002) peak of MoS 2 show significant intensities, which reflects incomplete exfoliation. However the ( 002) peaks vanish completely in the exfoliated Na-intercalated and Li-intercalated samples, which is a signature of complete exfoliation [29] , [30] . After annealing at 150 °C to remove water, weak ( 002 ) peaks recover in the Na and Li-exfoliated samples due to limited degree of restacking ( Supplementary Fig. S3 ). Solid-state NMR is used to study the local coordination environments of the alkali metal cations before and after hydration ( Fig. 2d,e ). The central peaks in freshly intercalated MoS 2 are sharp and symmetrical indicating a highly uniform chemical environment for most intercalated cations. After hydration, both central peaks of Li 7 and Na 23 solid NMR are broadened and shifted to lower frequencies, which can be attributed to dynamic processes or complex coordination environment with H 2 O molecules. Morphology characterization The uniformity and size distribution of the single-layer LTMDs sheets are examined using scanning electron microscopy (SEM) ( Fig. 3a,d ). One remarkable result is that 80% of the single-layer MoS 2 sheets has lateral widths of around 10 μm, this about 10 times larger than solution-exfoliated flakes reported using n -butyl lithium methods [28] , [30] . As shown in Fig. 3a , a typical single-layer MoS 2 flake has a surface area of 400 μm 2 . When the same intercalation-and-exfoliation process is performed on WS 2 crystals, 80% of the exfoliated flakes obtained are determined to be single layers with lateral dimensions between 3 and 10 μm, which essentially match the grain size of WS 2 powder before exfoliation ( Fig. 3d ). To assess the effectiveness of this method, the exfoliation yield in terms of micron-sized flakes is compared with the commonly used exfoliating agent n -butyl lithium on the same starting materials, the results show that only submicron-sized flakes can be generated using the latter ( Supplementary Figs S4–S6 ). 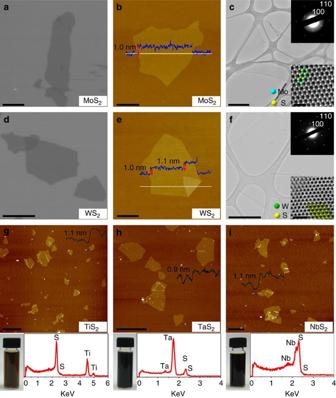Figure 3: Mophology characterization of LTMDs. (a) SEM images of Na-exfoliated single-layer MoS2. (b) AFM images of Na-exfoliated single-layer MoS2. (c) TEM images of Na-exfoliated single-layer MoS2, insets are the corresponding SAED and aberration-corrected HRTEM images. (d) SEM images of Na-exfoliated single-layer WS2. (e) AFM images of Na-exfoliated single-layer WS2. (f) TEM images of Na-exfoliated single-layer WS2, insets are the corresponding SAED and aberration-corrected HRTEM images. (g) AFM images TiS2, and corresponding EDS and photograph of dispersion in water. (h) AFM images of TaS2. (i) AFM images of NbS2. (g–i) give average thickness of ~1 nm, confirming that single-layer is successfully produced by our method. Scale bars in (a) is 10 μm, in (b,d,g,h) are 5 μm, in (c,e) are 1 μm, in (f) is 500 nm, in (i) is 2 μm, in inner images of (c,f) are 1 nm. Figure 3: Mophology characterization of LTMDs. ( a ) SEM images of Na-exfoliated single-layer MoS 2 . ( b ) AFM images of Na-exfoliated single-layer MoS 2 . ( c ) TEM images of Na-exfoliated single-layer MoS 2 , insets are the corresponding SAED and aberration-corrected HRTEM images. ( d ) SEM images of Na-exfoliated single-layer WS 2 . ( e ) AFM images of Na-exfoliated single-layer WS 2 . ( f ) TEM images of Na-exfoliated single-layer WS 2 , insets are the corresponding SAED and aberration-corrected HRTEM images. ( g ) AFM images TiS 2 , and corresponding EDS and photograph of dispersion in water. ( h ) AFM images of TaS 2 . ( i ) AFM images of NbS 2 . ( g – i ) give average thickness of ~1 nm, confirming that single-layer is successfully produced by our method. Scale bars in ( a ) is 10 μm, in ( b , d , g , h ) are 5 μm, in ( c , e ) are 1 μm, in ( f ) is 500 nm, in ( i ) is 2 μm, in inner images of ( c , f ) are 1 nm. Full size image The thickness of the exfoliated sheets is characterized by atomic force microscopy (AFM). Fig. 3b,e show typical tapping mode AFM images of exfoliated MoS 2 and WS 2 deposited on a SiO 2 /Si substrate by spin-coating. The average topographic height is around 1 nm, which agrees with typical height of a single-layer MoS 2 (between 0.6 and 1.0 nm) [30] . Statistical analysis of 100 flakes produced by the three different alkali metal adduct reveal 20, 90, and 80% of the flakes to be monolayer for K x MoS 2 , Na x MoS 2 , and Li x MoS 2 , respectively ( Supplementary Fig. S7 ). Although K x MoS 2 reacts more violently with water than Na x MoS 2 and Li x MoS 2 , its large ionic radius precludes full intercalation. Intercalating WS 2 with sodium naphthalenide also produces single-layer WS 2 flakes with a yield of~90%. Transmission electron microscopy (TEM) and selected area electron diffraction (SAED) were performed on the exfoliated flake suspended on a lacey carbon TEM grid ( Fig. 3c,f ). The SAED patterns of exfoliated MoS 2 and WS 2 exhibit high crystallinity (the inset in Fig. 3c,f , Supplementary Fig. S8 ), as judged from the characteristic honeycomb lattice. From XPS analysis, the Na-exfoliated MoS 2 film shows Mo 3 d peaks with peak position and width characteristic of the 2H phase [28] ( Supplementary Figs S9–S11 ). Optical characterization The Raman spectra of the exfoliated MoS 2 flakes were recorded using a 532-nm excitation line ( Fig. 4a and Supplementary Fig. S12 ). For Na-exfoliated samples, the E 1 2g phonons stiffen with decreasing number of layers and a blue shift of the peak from 380 cm −1 of the thick layers to 383 cm −1 of monolayer MoS 2 occurs. On the other hand, A 1g phonons soften with decreasing number layers, giving rise to a red shift from 407 cm −1 in the bulk material to 403 cm −1 in the monolayer. The Raman signature obtained is consistent with that of mechanically exfoliated single-layer MoS 2 (ref. 36 ). The corresponding Raman peaks in Li-exfoliated MoS 2 are much broader, which can be due to slight doping and possible presence of defects. 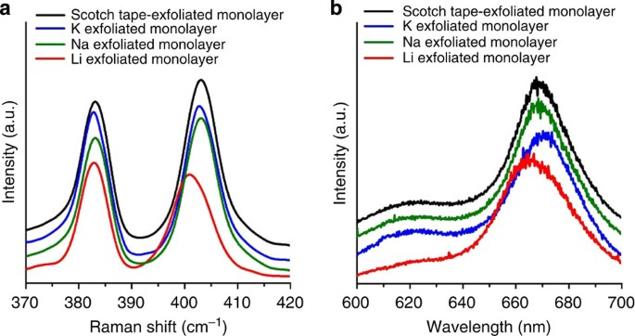Figure 4: Raman and photoluminescence spectrum of MoS2. (a) Raman spectra of scotch-tape-exfoliated single-layer MoS2and Na-, K- and Li-exfoliated single-layer MoS2deposited on Si/SiO2substrate. (b) Photoluminescence spectrum of scotch-tape-exfoliated single-layer MoS2, and Na-, K- as well as Li-exfoliated single-layer MoS2nanosheet deposited on Si/SiO2substrate. Figure 4: Raman and photoluminescence spectrum of MoS 2 . ( a ) Raman spectra of scotch-tape-exfoliated single-layer MoS 2 and Na-, K- and Li-exfoliated single-layer MoS 2 deposited on Si/SiO 2 substrate. ( b ) Photoluminescence spectrum of scotch-tape-exfoliated single-layer MoS 2 , and Na-, K- as well as Li-exfoliated single-layer MoS 2 nanosheet deposited on Si/SiO 2 substrate. Full size image Single-layer MoS 2 exhibits a unique signature in its optical spectrum in the form of photoluminescence (PL) due to the transition from an indirect to a direct-bandgap semiconductor ( Supplementary Fig. S13 ). MoS 2 appears in two distinct symmetry: 2H (trigonal prismatic D3h) and 1T (octahedral Oh) phases. The 2H phase is semiconducting while 1T is metallic ( Supplementary Note 1 ). In this work, PL can be observed on the exfoliated flakes after a brief bake at 200 °C to transform it to the 2H phase. As shown in Fig. 4b , the PL spectrum of a Na-exfoliated single-layer MoS 2 exhibits a peak centred at 668 nm (1.86 eV) with a shoulder at 623 nm (1.99 eV), which agrees with excitonic peaks arising from the K point of the Brillouin zone. The PL peak position and peak width is consistent with mechanically cleaved monolayer MoS 2 (ref. 3 ). The Li-exfoliated monolayer sample shows a weaker PL peak, this reflects either slight doping or the presence of defects in it. The chemical purity of the Na-exfoliated MoS 2 flakes is verified by energy-dispersive X-ray spectroscopy ( Supplementary Fig. S14 ) and its electrical property is evaluated in the form of a field effect transistor ( Supplementary Fig. S15 and Supplementary Note 2 ). The field effect mobility of monolayer MoS 2 flake is measured to be in the range of 1–8 cm 2 /(V × s)while that of few layer MoS 2 flakes are in the range of 20–80 cm 2 /(V × s), which are comparable with those of field effect transistor made from mechanically exfoliated MoS 2 flakes [37] . Inkjet printing Inkjet printing is highly promising for the high-throughput deposition of micron-sized patterns by virtue of its speed, low cost, additive and direct writing capability [38] . The good dispersion and high viscosity of our MoS 2 dispersion render it highly suitable for jet-printing. The ink is made from 0.02 mg ml −1 MoS 2 fully dispersed in ethanol/water (2:1 volume) solution (viscosity 2.64 cP and surface tension 34.3 mN m −1 ). To print high-resolution patterns and uniform films, 10-μm diameter printer nozzle is selected, and the wafers are heated to 60 °C before printing ( Supplementary Figs S16, S17 and Supplementary Note 3 ). Owing to the moderate surface energy of the ink, MoS 2 inks can be directly printed on plastic, SiO 2 , glass and optical fibre pigtail ( Fig. 5a–d ) without any chemical/physical modification. 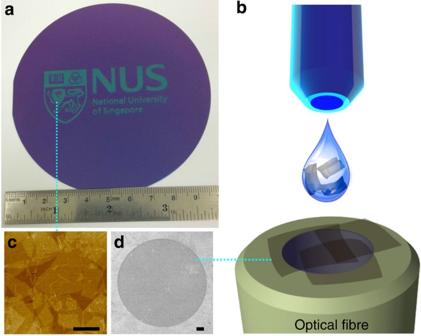Figure 5: Inkjet printing of MoS2. (a) Wafer-scale MoS2pattern jet-printing. Large area, continuous and highly uniform MoS2thin film pattern were directly printed on a 4-inch Si/SiO2wafer by inkjet printing. (b) Schematic showing the printing of MoS2thin film on the optical fibre pigtail. (c) AFM image of MoS2thin film, showing a thickness of 1–4 layers. (d) SEM image of MoS2thin film-coated optical fibre pigtail. Scale bar is 5 μm in (c,d). Figure 5a shows the word ‘NUS’ printed directly using the MoS 2 flakes. The AFM and SEM characterization of the MoS 2 printed thin film show that the printed MoS 2 film is continuous and uniform with a sheet thickness of 2–3 layers, as shown in Fig. 5c,d . Figure 5: Inkjet printing of MoS 2 . ( a ) Wafer-scale MoS 2 pattern jet-printing. Large area, continuous and highly uniform MoS 2 thin film pattern were directly printed on a 4-inch Si/SiO 2 wafer by inkjet printing. ( b ) Schematic showing the printing of MoS 2 thin film on the optical fibre pigtail. ( c ) AFM image of MoS 2 thin film, showing a thickness of 1–4 layers. ( d ) SEM image of MoS 2 thin film-coated optical fibre pigtail. Scale bar is 5 μm in ( c , d ). Full size image In summary, we have explored the use of metal naphthalenide for the intercalation–exfoliation of metal chalcogenides (MoS 2 and WS 2 ) and obtained high-efficiency exfoliation of micron-sized monolayer sheet (widths in the range of 5–10 μm). The size distribution of the flake is much better than exfoliation using organolithium salts ( n -butyl lithium). This can be related to a reduced chemical reaction of the radical anion (C 10 H 8 − ) with the host material, and the fact that we apply a pre-expansion procedure with hydrazine to facilitate the efficient intercalation of the metal cations. Evidence from XRD and NMR shows the existence of highly ordered ternary phase after cation intercalation. In terms of exfoliation efficiency, sodium naphthalenide (Na + C 10 H 8 − ) produces higher quality monolayer flake than its lithium and potassium counterparts. This work contributes a high-yield chemical processing method for producing high-quality 2D chalcogenide monolayers with direct relevance to printable photonics. Pre-expansion of MoS 2 Bulk MoS 2 (1.6 g; SPI, single crystal) and 20 ml hydrazine hydrate (Aldrich, 98%) are sealed in an autoclave and heated at 130 °C for 48 h. The expanded MoS 2 , which has a worm-like appearance, is washed three times by water and dried at 120 °C for 10 h. Intercalation of MoS 2 Na (0.69 g; Aldrich) (for K or Li, we used 1.08 g or 0.21 g, respectively), 1.92 g naphthalene (aldrich) and 80 ml anhydrous tetrahydrofuran (THF) (Aldrich, fresh redistilled by Na) are stirred for 2 h in ice-water bath in argon atmosphere. Pre-expanded MoS 2 powder (1.6 g) is added to the dark blue solution and the mixture is further stirred for 5 h. After reaction, the product is washed five times by anhydrous THF. The procedures are similar for both K and Li. Intercalation process for WS 2 is similar except that 2.48 g of WS 2 is used with the same amount of reagent above. Caution: Li x MoS 2 will self-heat in air, Na x MoS 2 will self-ignite in air and K x MoS 2 will self-explode in air. Exfoliation Distilled water (100 ml) is added to the intercalated sample. The mixture is sonicated in a low-power sonic bath (60 W) for 30 min to form a homogeneous suspension. The mixture is centrifuged at 8,000 r.p.m. for 15 min for several cycles to remove excess impurity, and then at 1,000 r.p.m. for 15 min in the last cycle. Equipment The following equipment were used: Raman (Alpha 300R), PL (equipped on Raman), SEM (Jeol JSM-6701F), AFM (Dimension Fast Scan), XPS (SPECS), UV-VIS-NIR (Shimadzu UV-3600), solid NMR (Bruker 400 MHz), powder XRD (Siemens D5005), Jet-Printer (Dimatix, 2800). How to cite this article: Zheng, J. et al. High yield exfoliation of two-dimensional chalcogenides using sodium naphthalenide. Nat. Commun. 5:2995 doi: 10.1038/ncomms3995 (2014).